High spectral resolution of gamma-rays at room temperature by perovskite CsPbBr3single crystals Gamma-ray detection and spectroscopy is the quantitative determination of their energy spectra, and is of critical value and critically important in diverse technological and scientific fields. Here we report an improved melt growth method for cesium lead bromide and a special detector design with asymmetrical metal electrode configuration that leads to a high performance at room temperature. As-grown centimeter-sized crystals possess extremely low impurity levels (below 10 p.p.m. for total 69 elements) and detectors achieve 3.9% energy resolution for 122 keV 57 Co gamma-ray and 3.8% for 662 keV 137 Cs gamma-ray. Cesium lead bromide is unique among all gamma-ray detection materials in that its hole transport properties are responsible for the high performance. The superior mobility-lifetime product for holes (1.34 × 10 −3 cm 2 V −1 ) derives mainly from the record long hole carrier lifetime (over 25 μs). The easily scalable crystal growth and high-energy resolution, highlight cesium lead bromide as an exceptional next generation material for room temperature radiation detection. High performance, low cost nuclear radiation detectors based on compound semiconductors are a highly sought technology over many decades because of their broad potential applications in the fields of homeland security (nonproliferation of nuclear materials), industrial and medical imaging, and fundamental scientific research [1] , [2] , [3] . For such applications, gamma rays (γ-rays) must be detected with high-spectroscopic resolution to discriminate the characteristic γ-ray spectrum used to identify radionuclides contained in the source. There are two main detection modes for γ-ray radiation, optical-based scintillators and electronic-based semiconductors. Compared to scintillation detectors, which suffer from the intrinsic nonproportionality of the light yield making it challenging to measure accurate γ-ray energies, the output pulse height from on a semiconductor detector is just proportional to the charge that is induced over a specific time interval and thus has superior accuracy in energy resolution [4] , [5] . Therefore, the quest for semiconductor materials for low cost effective radiation detectors has existed from the dawn of the semiconductor era and persists to the present date [6] . Prospective semiconductors need to fulfill simultaneously several desirable properties. The detector material should be: capable of interacting strongly with the high-energy photons; operable under high electric field with negligible leakage current; allowing for the photo-generated carriers to drift through the detector volume unimpeded, this means they must have extremely low concentration of charge trapping and electrically active defects; and must be easily upscalable to low cost [7] . On this premise, only few inorganic compounds, specifically Cd 1− x Zn x Te (CdZnTe), CdTe, TlBr, and α-HgI 2 , are able to combine some of the above-mentioned characteristics and demonstrate a spectroscopic response [1] , [8] , [9] , [10] , [11] . However, each suffers from persistent unsolved issues associated with difficulties encountered in the crystal growth or in device operation [1] , [12] , [13] . For instance, secondary phases are always present in detector-grade CdZnTe crystals, such as inclusions and precipitates, and can degrade the local charge transport properties and the uniform response of detectors [14] , [15] . From the above compounds only CdZnTe, which has been in continuous development since the 1970s, has been commercialized for room temperature applications, albeit it at a high cost that limits widespread use. Since 2012, halide perovskites with a general formula of AMX 3 , where A + = Cs, CH 3 NH 3 , HC(NH 2 ) 2 , M 2+ = Ge, Sn, Pb, and X − = Cl, Br, I, have attracted intense interest because of facile synthesis and processing, as well as impressive optical and electronic properties, such as an extremely low density of defects, excellent carrier transport, and surprisingly high defect tolerance [16] , [17] , [18] , [19] , [20] , [21] . However, in general, organic–inorganic hybrid perovskites intrinsically have structural disorder in the strongly polar organic cations and structurally dynamic inorganic frameworks, causing long-term chemical instability [18] , [20] , [22] . The all-inorganic perovskite CsPbBr 3 features a favorable electronic structure with a large bandgap of 2.3 eV, broad valence and conduction bands and can grow in large crystal sizes from its melt, as well as from solution. It also offers far greater long-term stability because it lacks organic molecules [23] , [24] , [25] , [26] , [27] . Furthermore, CsPbBr 3 is a high Z compound with effective atomic number Z eff of 65.9, which is much higher than CdZnTe (50.2). 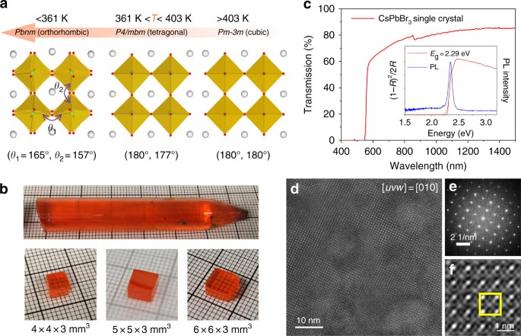Fig. 1 Crystal growth and general properties of CsPbBr3.aNondestructive phase transitions in CsPbBr3during cooling involving small rotations and tilts of PbBr6octahedral (associated with anglesθ1andθ2). The Cs, Pb, and Br atoms are depicted as gray, green, and red spheres, respectively.bAs-grown single crystal ingot with a diameter of 11 mm, and the single crystal wafers with different sizes, 4 × 4 × 3 mm3, 5 × 5 × 3 mm3, and 6 × 6 × 3 mm3. The smallest grid size corresponds to 1 mm. The pure orthorhombic phase of the crystal was confirmed by powder X-ray diffraction in Supplementary Figure2.cOptical transmission spectrum for CsPbBr3single crystals with size of 5 × 5 × 3 mm3. Insets are the optical absorption spectrum obtained from diffuse reflectance measurement on ground CsPbBr3crystals and the steady-state PL of CsPbBr3single crystal excited at 440 nm.dHigh resolution TEM (HRTEM) with selected area electron diffraction (SAD) ine, and magnified lattice image inf. Yellow squares infare drawn to compare HRTEM image and simulations in Supplementary Figure3 Thus, the attenuation coefficients of CsPbBr 3 for γ-rays are higher than CdZnTe, leading to even higher stopping power especially in the high energy region (100–500 keV, Supplementary Figure 1 ). We initiated our research on CsPbBr 3 in 2013 as a potential hard radiation detector material [23] . However, our previous and subsequent works did not yet deliver the detection of highly resolved γ-rays [24] , [25] , [26] . Here we report a modified melt growth method for CsPbBr 3 , which results in very high purity material capable of detecting γ-rays as we demonstrate with 57 Co 122 keV and 137 Cs 662 keV γ-rays (as well as 22 Na and 241 Am γ-rays). In addition to achieving high crystal quality of CsPbBr 3 , we accomplish this by applying a special device architecture that dramatically reduces the leakage current under large electric field. We have thus produced CsPbBr 3 planar detectors reproducibly, which show the best spectral resolution (3.8–3.9%) obtained for any halide perovskite and non-perovskite material to date and comparable to commercial samples of the benchmark CdZnTe planar detector which gives 4.1% for with 57 Co 122 keV but can hardly resolve the 662 keV 137 Cs γ-rays [28] . Improved single crystal growth CsPbBr 3 exhibits two nondestructive phase transitions at relatively low temperatures. The first phase transition which occurs around 130 °C from cubic ( Pm-3m ) to tetragonal ( P4/mbm ) is a first-order phase transition. This is followed by a second order transition around 88 °C to the orthorhombic ( Pbnm ) phase, which is stable at room temperature, Fig. 1a [23] . Such phase transitions can induce residual stress or mechanical deformations and can lead to the formation of cracks or sub-grain boundaries or twins. Those structural defects could be detrimental to detector performance, and thus should be mitigated as much as possible during crystal growth. Fig. 1 Crystal growth and general properties of CsPbBr 3 . a Nondestructive phase transitions in CsPbBr 3 during cooling involving small rotations and tilts of PbBr 6 octahedral (associated with angles θ 1 and θ 2 ). The Cs, Pb, and Br atoms are depicted as gray, green, and red spheres, respectively. b As-grown single crystal ingot with a diameter of 11 mm, and the single crystal wafers with different sizes, 4 × 4 × 3 mm 3 , 5 × 5 × 3 mm 3 , and 6 × 6 × 3 mm 3 . The smallest grid size corresponds to 1 mm. 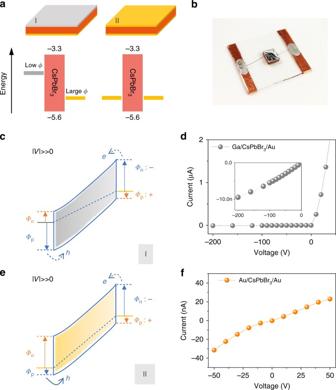Fig. 2 Architecture and electrical properties for CsPbBr3detectors.aI and II depict two different designs with asymmetrical and symmetrical electrode materials, and their corresponding energy level diagrams.bTypical high performance Ga/CsPbBr3/Au detector.c,eBand diagrams of two different CsPbBr3detectors under large reversed electric fields. Note that the “+,” “−” andΦnandΦprepresent the forward and reversed bias and Schottky barrier for electron and hole at the semiconductor–metal interface, respectively.d,fTypicalI–V characteristic curve of the Type I (Ga/CsPbBr3/Au) and Type II (Au/CsPbBr3/Au) detectors The pure orthorhombic phase of the crystal was confirmed by powder X-ray diffraction in Supplementary Figure 2 . c Optical transmission spectrum for CsPbBr 3 single crystals with size of 5 × 5 × 3 mm 3 . Insets are the optical absorption spectrum obtained from diffuse reflectance measurement on ground CsPbBr 3 crystals and the steady-state PL of CsPbBr 3 single crystal excited at 440 nm. d High resolution TEM (HRTEM) with selected area electron diffraction (SAD) in e , and magnified lattice image in f . 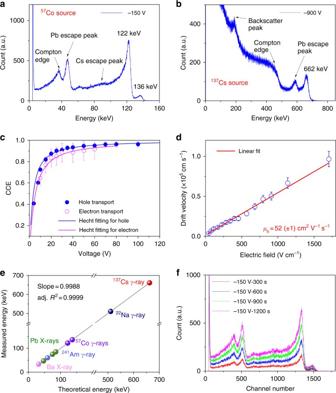Fig. 3 γ-ray response of Type I CsPbBr3detectors to different radioactive isotopes.aEnergy-resolved spectrum of57Co γ-ray source with a characteristic energy of 122 keV using a shaping time of 2 μs. The dimension of the detector is 3 × 3 × 0.90 mm3.bEnergy-resolved spectrum of137Cs γ-ray source with the characteristic energy of 662 keV with a shaping time of 0.5 μs. The dimension of the detector is 4 × 2 × 1.24 mm3.cThe mobility-lifetime fitting for electron and hole according to the Hecht equation based on the spectra indicated in Supplementary Figure7. The error bars in CCE arising from obtaining the peak/shoulder channel number represent ±3% and ±10% errors for hole and electron, respectively.dHole mobilityμhof CsPbBr3evaluated from the rise time distribution versus applied bias according to the equationμ=d2/(tr×V), where thed,tr, andVare the detector thickness, the rise time, and applied voltage, respectively. The drift velocity is calculated asd/tr. The distribution histogram for corresponding rise time is indicated in Supplementary Figure12. The error bars in carrier drift velocity represent ±10% errors arising from obtaining rise time.eHighly linear detection response of CsPbBr3planar detectors to different radiation sources and the corresponding spectra are shown in Supplementary Figure10.fThe stability of spectrum of CsPbBr3detector over a period of 20 min under57Co γ-source measured with a shaping time of 2 μs and applied voltage of −150 V Yellow squares in f are drawn to compare HRTEM image and simulations in Supplementary Figure 3 Full size image One of the dramatic improvements achieved in this work is the optimization of our crystal growth process that can produce large crack-free single crystal ingots with diameter of 11 mm and length over 6 cm (Fig. 1b ). We stress that the detailed kinetic parameters during the crystal growth process are extremely important. The melt temperature, temperature gradient, and cooling strategies are critical and have been optimized over multiple growth runs. The single crystal ingot in Fig. 1b was grown with a slow translation velocity of 0.5 mm h −1 with the specific overheating temperature and temperature gradient of 15 K and 9 K cm −1 , respectively. The cooling strategy is particularly important for avoiding structural defects due to the low temperature phase transitions. The translation speed after crystallization was to keep the cooling rate very low at about 5 K h −1 and produced an orange-red transparent single crystal ingot free of visible cracks or grain boundaries. Supplementary Figure 4 illustrates the sensitivity of single crystal CsPbBr 3 to the growth parameters by comparing the transmission spectra and detector performance of crystals grown with suboptimal growth speeds and cooling rates. The ingot was then cut and fabricated into wafers with regular shapes for detectors. Compared to solution growth in organic solvents [25] , crystal growth from melt has significant advantages, such as control and amenability to scale-up. Moreover, melt growth under vacuum conditions inhibits the unintended contamination from solutions leading to higher purity level and better crystalline quality. The impurity levels in our CsPbBr 3 single crystals, for up to 69 elements, were analyzed by the glow discharge mass spectrometry technique and their concentrations are listed in Supplementary Table 1 . The total-impurity concentration for all elements is below 10 p.p.m. The impurities with concentration above 0.5 p.p.m. are Rb (1.3 p.p.m. ), Ca (0.72 p.p.m. ), Cl (6.8 p.p.m. ), and I (less than 0.8 p.p.m. ), which consist of over 90% of the total-impurity concentration. Those impurities are highly miscible with CsPbBr 3 and likely incorporated from the precursor materials. These results confirm that the CsPbBr 3 single crystal is highly chemically pure. The optical transmittance for a 3 mm thick crystal exceeded 65% when the wavelength was over 600 nm and exceeded 80% when over 1000 nm (Fig. 1c ). The high transmittance indicates that the as-grown single crystals do not have any significant concentration of optical absorption or scattering centers below the bandgap energy of 2.29 eV. The steady-state photoluminescence (PL) for our CsPbBr 3 single crystal corresponds well to the previously observed bound exciton emission [29] at 2.34 eV, while the time-resolved photoluminescence (TRPL) indicated biexponential decay (Supplementary Figure 2 and Supplementary Note) with a rapid component (19 ± 13 ns) and a slower component (122 ± 13 ns). The decay time in our crystals is significantly longer than in crystals grown from solution methods, indicating fewer traps and higher crystalline quality [30] . High resolution transmission electron microscopy (HRTEM) was used to further investigate structural uniformity on the atomic and nano scale (Supplementary Note). A cross-sectional TEM sample was prepared parallel to the edge of the cleaved plane using focused ion beam technology as illustrated in Supplementary Figure 3 . Single crystallinity and excellent uniformity of CsPbBr 3 was confirmed using selected area diffraction and HRTEM with FFT. The zone axis of HRTEM in Fig. 1d is determined to be the [010] zone based on the TEM image simulation. No precipitates were found in the as-grown single crystals. Asymmetric electrode design For planar CsPbBr 3 -based hard radiation detectors there are two basic types, Type I and Type II, as illustrated in Fig. 2a . Type I configuration involves an asymmetric choice of detector electrodes where one metal has low work function and the other high, while Type II replies on identical electrodes on both sides of the crystal. Here we demonstrate the efficacy of the Type I structure in fabricating efficient planar radiation detectors. The as-grown CsPbBr 3 single crystals show p- type behavior as judged from the positive Seebeck coefficient, S (300 K) = +723(±45) μV K −1 , at room temperature. To illustrate the energy level diagram in Fig. 2a , we consider that the conduction band minimum and valence band maximum in CsPbBr 3 are at −3.3 and −5.6 eV, respectively. These energy levels and the p -type behavior of the material need to be taken into account in choice of electrodes [31] . Typical high work function electrode metals/materials are Au and Pt but can also be organic or inorganic hole extraction layers (HELs). Low work function metals/materials are usually Al, Ga, and In, but also organic or inorganic electron extraction layers. Fig. 2 Architecture and electrical properties for CsPbBr 3 detectors. a I and II depict two different designs with asymmetrical and symmetrical electrode materials, and their corresponding energy level diagrams. b Typical high performance Ga/CsPbBr 3 /Au detector. c , e Band diagrams of two different CsPbBr 3 detectors under large reversed electric fields. Note that the “+,” “−” and Φ n and Φ p represent the forward and reversed bias and Schottky barrier for electron and hole at the semiconductor–metal interface, respectively. d , f Typical I –V characteristic curve of the Type I (Ga/CsPbBr 3 /Au) and Type II (Au/CsPbBr 3 /Au) detectors Full size image Based on the Type I design, we devised an effective electrode configuration for CsPbBr 3 detectors that can dramatically reduce the dark current by at least three orders of magnitude, while providing impressive temporal stability, especially under high electric field. Ga metal with its relatively small work function ( ϕ Ga 4.3 eV) was chosen to form a higher Schottky barrier potential Φ p under reversed bias. Other materials, such as Al ( ϕ Al 4.1 eV) and In ( ϕ In 4.1 eV) and organic HELs, also work similarly without a significant change in energy spectrum. Therefore, for simplicity, we only discuss Ga/CsPbBr 3 /Au detector (Fig. 2b ). The assortment of the energy diagram for this metal–semiconductor–metal system generates both higher Schottky barriers Φ n and Φ p at the semiconductor–metal interface as the device is reversely biased, Fig. 2c . For such a device, the characteristic I – V curve in Fig. 2d and Supplementary Figure 5a is sublinear and superlinear in the negative and positive voltage range, respectively, owing to deficient injection under reverse bias and excessive injection under forward bias [32] . Even under very large negative bias (−200 V, corresponding to 2000 V cm −1 ), the leakage current is also kept small, around −10 nA (corresponding to 83.3 nA cm −2 , Fig. 2d ). In comparison, as indicated in Supplementary Figure 5c , under higher bias (200 V, 2000 V cm −1 ) the Type II device shows a considerable dark current over 100 μA, corresponding a current density of 1.1 × 10 6 nA cm −2 , which is over 10 4 times higher than that of Type I device. In addition, the dark current of the Type I device is very stable with time, the corresponding I – t curve is shown in Supplementary Figure 5b . Overall, the greatly suppressed dark current results in lower detector operation noise. Another great feature of the Type I detector is that the Au electrode is serving as the charge collection contact, which can also be advantageous in the fabrication technologies of pixelated or coplanar-grid detectors from the current CdZnTe technology [33] . The energy diagram for the symmetric Type II electrode configuration under high electric field is depicted in Fig. 2e . In this case, owing to the smaller Schottky barrier Φ p at the metal–semiconductor junction holes can be easily injected into the crystal from the positive electrode through tunneling or thermionic emission mechanism [34] given the p -type character of CsPbBr 3 . This can contribute to a large dark leakage current (Fig. 2f ). Particularly under high electric field (over 1000 V cm −1 ) for Type II detector the leakage current is usually on the order of microamperes (Supplementary Figure 5c ). In addition, the leakage current under high electric field continuously increases over time as extra holes are injected into the system (Supplementary Figure 5d ), a temporal instability which prevents the Type II planar detector’s use as a stable and effective γ-ray detector. The resulting background noise from the leakage current of the detector will ruin the energy resolution of the spectrum and the typical γ-ray spectra obtained from the Type II detector will be ill defined at best (Supplementary Figure 6 ). γ-ray spectral performance Under a 59.5 keV 241 Am γ-ray source (Supplementary Figure 7a ), Type I device (Ga/CsPbBr 3 /Au) showed well-resolved spectroscopic response with the full width at half maximum (FWHM) in percentage of 9.6(±0.5)%. The applied voltage (−150 V, corresponding to a field of 1667 V cm −1 ) and the induced charge Q collection were both on the Au cathode, while the γ-ray irradiated Ga anode was grounded. Thus, the measured signal is generated mainly by holes drifting through the entire thickness of the detector. Distinct charge transport properties for electron and hole collection modes are shown in Supplementary Figure 7 . When exposed to a 0.2 mCi 57 Co γ-ray source with a characteristic energy of 122 keV, the CsPbBr 3 detector also delivered a series of excellent 57 Co γ-ray spectra with extremely low contribution from leakage current noise (Fig. 3a and Supplementary Figure 8 ) and achieves an energy resolution by FWHM of 4.3(±0.2)% under −150 V. The above results were obtained reproducibly and also confirmed by measurements at Fisk University, where a slightly better energy resolution of 3.9(±0.2)% under −150 V was obtained for the CsPbBr 3 detector (Supplementary Figure 9 ). Exposure of our detector to a 5 µCi 137 Cs source with characteristic energy of 662 keV yielded, as well-resolved spectrum with an energy resolution of 3.8(±0.2)%, see Fig. 3b . The CsPbBr 3 detector also resolved the spectral line of 22 Na at 511 keV (Supplementary Figure 10 ). Such high resolution is in fact comparable to a commercial reference CdZnTe planar detector tested under the same experimental conditions, which demonstrated FWHM of 4.1% for 57 Co (Supplementary Figure 8 ) but poorly resolved the 662 keV of 137 Cs [28] . Indeed, CZT detectors equipped with special contact designs and pulse discrimination, pixelated designs and proper ASIC readout electronics can dramatically improve the energy resolution to a higher level for 662 keV of 137 Cs to about 1% [35] . Fig. 3 γ-ray response of Type I CsPbBr 3 detectors to different radioactive isotopes. a Energy-resolved spectrum of 57 Co γ-ray source with a characteristic energy of 122 keV using a shaping time of 2 μs. The dimension of the detector is 3 × 3 × 0.90 mm 3 . b Energy-resolved spectrum of 137 Cs γ-ray source with the characteristic energy of 662 keV with a shaping time of 0.5 μs. The dimension of the detector is 4 × 2 × 1.24 mm 3 . c The mobility-lifetime fitting for electron and hole according to the Hecht equation based on the spectra indicated in Supplementary Figure 7 . The error bars in CCE arising from obtaining the peak/shoulder channel number represent ±3% and ±10% errors for hole and electron, respectively. d Hole mobility μ h of CsPbBr 3 evaluated from the rise time distribution versus applied bias according to the equation μ = d 2 /( t r × V ), where the d , t r , and V are the detector thickness, the rise time, and applied voltage, respectively. The drift velocity is calculated as d / t r . The distribution histogram for corresponding rise time is indicated in Supplementary Figure 12 . The error bars in carrier drift velocity represent ±10% errors arising from obtaining rise time. e Highly linear detection response of CsPbBr 3 planar detectors to different radiation sources and the corresponding spectra are shown in Supplementary Figure 10 . f The stability of spectrum of CsPbBr 3 detector over a period of 20 min under 57 Co γ-source measured with a shaping time of 2 μs and applied voltage of −150 V Full size image The carrier mobility and mean free drift time (lifetime) product, µτ , is extracted from the voltage dependence of the charge collection efficiency (CCE) according to the Hecht equation [36] from the spectroscopic voltage dependence data for holes and electrons are 1.34 × 10 −3 and 8.77 × 10 −4 cm 2 V −1 , respectively (Fig. 3c ). The µτ values for holes and electrons are comparable. This is a unique feature among γ-ray detector materials and is a major advantage for the fabrication of simple detectors. The hole mobility-lifetime product values for our CsPbBr 3 crystals are one or two orders of magnitude higher than that of the benchmark CdTe and CdZnTe materials, ( µτ ) h approximate 10 −4 –10 −5 cm 2 V −1 , and is comparable to their ( µτ ) e which ranges from 10 −3 to 1 × 10 −2 cm 2 V −1 13 . We evaluated the hole mobility of our CsPbBr 3 crystals based on the distribution of rise times t r extracted from the transient pulses generated by 241 Am γ-ray, as has been commonly applied for CdTe and CdZnTe materials [37] . The hole mobility of 52(±1) cm 2 V −1 s −1 was obtained which is also consistent with the theoretical polaron hole mobility, 41.3 cm 2 V −1 s −1 , for CsPbBr 3 [38] . The experimental mobility-lifetime product, µτ , and hole mobility, µ , obtained above give an unprecedented long lifetime τ for holes of about 25 μs. This strikingly long lifetime is longer than all known radiation detection compound semiconductors. In addition, this is an unprecedented example of a high-spectral resolution γ-ray detecting semiconductor with better hole transport properties than electron transport properties. The presence of strong carrier–phonon coupling in CsPbBr 3 is a consequence of the dynamic disorder in the perovskite structure [39] , and thus we surmise it contributes to the surprisingly long lifetimes observed. To determine the spectral linearity of the CsPbBr 3 detector, we obtained an energy-calibrated spectrum according to the photopeak position of 57 Co γ-ray (122 keV). A series of photopeaks from different radioactive isotopes are clearly resolved (Supplementary Figure 10 ) at 32.3 keV (Ba X-ray), 47 keV (Pb escape X-ray), 75 and 85 keV (Pb characteristic X-rays from shielding material used), 59.5 keV ( 241 Am γ-ray), 122 and 136 keV ( 57 Co γ-ray), 511 keV ( 22 Na γ-ray), and 662 keV ( 137 Cs γ-ray). As shown in Fig. 3e , the linear (or proportionality) response of such device is excellent, over 0.99. In addition, we also performed an experiment for further demonstration of the simultaneous discrimination of different radioisotopes under identical conditions, as indicated in Supplementary Figure 11 . Moreover, the average ionization energy ( ε pair ) defined by the average minimum energy required to ionize an electron–hole pair in CsPbBr 3 is determined to be around 5.3 eV (Supplementary Figure 13 ). Our CsPbBr 3 detector has demonstrated excellent stable response over time. Over a continuous operation period of 1200 s, the peak channel number, count rate (counts per second) and FWHM for 57 Co γ-ray spectrum were unchanged (Fig. 3f and Supplementary Figure 14 ), confirming that polarization induced by charge trapping is surprisingly absent for devices with Type I design. The feature of high defect tolerance and low impurity concentration in the CsPbBr 3 crystals likely play an important role in suppressing polarization under detector operating conditions. The super-long hole lifetime (25 μs) is good evidence for lacking deep-level traps, which will in general substantially reduce the carrier drift lifetime. Thermally stimulated current (TSC) spectroscopy (Supplementary Figure 15 and Supplementary Note) for our CsPbBr 3 single crystals further confirmed the very low trap density (between 4.11 × 10 14 cm −3 and 5.29 × 10 15 cm −3 ) and lack of deep-level defects. As indicated in Supplementary Table 2 , only five traps with energy level below 0.28 eV were identified. A relatively long-term detection operation test was also carried out and the CsPbBr 3 detector demonstrated excellent stability by a continuous operation period over 120 h with the same count rate was retained, while the channel number of the 57 Co γ-ray photopeak was reduced slightly by 3.4% (Supplementary Figure 16 ). Detector performance of CsPbBr 3 detectors fabricated from different batches of crystals grown under the same growth conditions have demonstrated highly resolved spectral peaks under 57 Co γ-ray irradiation reproducibly (Supplementary Figure 17 ). The robustness and reproducibility of the crystal growth and device design could definitely push the CsPbBr 3 to the leading room temperature radiation detection material considering the promise of low cost, easy scale-up and high performance (Supplementary Table 3 ). In conclusion, we demonstrated the high resolution γ-ray detection response from high-quality perovskite CsPbBr 3 perovskite single crystals. We obtained crack free, large single crystal ingots with very high purity (below 10 p.p.m. of total impurities) and low defect density using an optimized scaled-up growth method. Deploying a special device design with asymmetrical electrode materials effectively suppresses the dark leakage current under high electric field and enables the CsPbBr 3 planar detectors to achieve remarkable energy resolving capabilities. Specifically, the CsPbBr 3 detector resolved the 59.5 keV ( 241 Am γ-ray), 122 and 136 keV ( 57 Co γ-ray), 511 keV ( 22 Na γ-ray), and 662 keV ( 137 Cs γ-ray) lines with best spectral resolution of 3.8%. This high performance is achieved by an unprecedentedly long hole lifetime (over 25 μs) and a superior mobility-lifetime product for holes (1.34 × 10 −3 cm 2 V −1 ). Furthermore, CsPbBr 3 detectors demonstrate long-term stability without observable significant polarization. Because of these promising properties (easy scale-up, low cost and high performance), we believe CsPbBr 3 is an exceptionally viable candidate for next generation room temperature radiation detectors and possibly displace the leading but problematic materials CdZnTe and TlBr. Materials Chemicals in this work were used as obtained: Cesium bromide, 99.999%, Sigma-Aldrich; Lead bromide, 99.999%, Sigma-Aldrich. Bridgman growth of CsPbBr 3 from its melt Polycrystalline CsPbBr 3 was prepared directly from CsBr and PbBr 2 by a solid-state reaction with a 1:1 stoichiometric ratio at 580 °C. For a small scale (less than 40 g), the synthesis and growth were done in the same fused silica tube to reduce unintended contamination that might occur in multistep process. The silica tube for Bridgman growth was of 11 mm inner diameter with a conical shaped end. All processes for synthesis and crystal growth were done in vacuum, with an original pressure less than 10 −4 Torr (at room temperature). The sealed silica tube was placed on a support rod, which moved downwards with a geared translation system inside a two-zone vertical furnace for single crystal growth. The silica tube was heated up to 590 °C in 10 h and held at that temperature for 12 h for overheating to avoid heterogeneous nucleation. A temperature of 15–30 K of melt overheating helps to reduce excess nucleation centers and suppress the formation of structural defects. The temperature profile was also optimized to avoid thermal-induced cracks and possible constitutional supercooling, thereby enhancing the single crystal yield of CsPbBr 3 . Once the silica tube completely passed with a dropping speed of 0.5–2 mm h −1 through the temperature gradient region (with a typical temperature gradient of 5–20 K cm −1 ), the ingot was cooled down to 200 °C in 20 h. Owing to the existence of phase transitions, the ingot was then cooled down to room temperature with a cooling rate of 2–5 K h −1 . It should be noted that excessive temperature gradient and dropping speed and cooling rate likely result in cracks and final fracture of the ingots (Supplementary Figure 4 ). Sample processing The CsPbBr 3 crystal ingots were cut into circular wafers perpendicular to the growth direction and to desired shapes of 0.5–2 mm thickness using a Struers Accutom-50 waferizing saw equipped with a 300 µm wide diamond-impregnated blade. The sample surfaces were then polished mechanically with successively fine SiC grinding papers down to 1 µm particle size. Electrode preparation The polished CsPbBr 3 crystals were rinsed in toluene to remove any possible surface contamination before the electrode deposition. The Au electrode was prepared by either brushing Au paint or thermal evaporation through a shielding mask onto CsPbBr 3 samples (30–100 nm thickness for evaporation). For the Ga electrode, it was simply prepared by brushing liquid Ga metal on the surface of the crystal. The electrodes were connected by Cu wire to the outer collection circuit. Electrical properties and detector performance measurements The I – V characteristic curves were measured by a Keithley 6517B electrometer under dark condition, where resistivity was calculated in the low bias range of −1 to 1 V. For detector performance measurements, the γ-ray sources employed were 1 µCi 241 Am 59.5 keV, 0.2 mCi 57 Co 122 keV, 50 µCi 22 Na 511 keV, and 5 μCi 137 Cs 662 keV γ-rays. eV-550 preamplifier with bias supply ranging from 4 to 1000 V (or −4 to −1000 V) was connected to the detectors placed in a shielding box. Note that voltage was applied to the bottom contact while the top contact was irradiated with γ-rays. The signal processing and generation of the γ-ray spectrum was described in our previous work [40] . The mobility-lifetime product ( μτ ) was calculated according to the Hecht equation [36] , [40] , \(\eta = \frac{Q}{{Q_0}} = \mu \tau \frac{V}{{d^2}}(1 - \mathrm{e}^{ - \frac{{d^2}}{{\mu \tau V}}})\) , where η is the CCE, Q and Q 0 is the maximum and theoretical saturated channel number of photopeak/shoulder, respectively, V is applied bias and d is the thickness of the detector. The mobility was estimated using pulse height spectroscopy [40] . We used the average rise time based on the distribution of rise times under each bias to estimate the mobility. Data availability The data that support the findings of this study are available from the corresponding author upon reasonable request.